Coordination and fine motor control depend onDrosophilaTRPγ Motor coordination is broadly divided into gross and fine motor control, both of which depend on proprioceptive organs. However, the channels that function specifically in fine motor control are unknown. Here we show that mutations in trpγ disrupt fine motor control while leaving gross motor proficiency intact. The mutants are unable to coordinate precise leg movements during walking, and are ineffective in traversing large gaps due to an inability in making subtle postural adaptations that are requisite for this task. TRPγ is expressed in proprioceptive organs, and is required in both neurons and glia for gap crossing. We expressed TRPγ in vitro , and found that its activity is promoted by membrane stretch. A mutation eliminating the Na + /Ca 2+ exchanger suppresses the gap-crossing phenotype of trpγ flies. Our findings indicate that TRPγ contributes to fine motor control through mechanical activation in proprioceptive organs, thereby promoting Ca 2+ influx, which is required for function. Even the most basic tasks, such as acquiring food, locating safe places to rest, avoiding and defending against enemies, and mating requires motile animals to navigate through their environment by moving multiple body parts in a highly coordinated manner. To move fluidly, both vertebrate and invertebrate animals employ complex mechanosensory organs that are designed to gather and interpret feedback information about their movement in real time through an array of specialized receptors and neural networks [1] , [2] . These proprioceptive sensory systems provide animals with continuously updated maps of their body positions that are critical for balance and locomotion. Proprioception is mediated at the cellular level, by stretch-sensitive cells located in muscles, ligaments and joints, which are activated by mechanical forces [3] , [4] , [5] . In humans, damage to proprioceptive afferents results in a variety of movement disorders such as spasticity, impaired load sensitivity, and altered gait [6] . Proprioceptive dysfunction is also a clinical feature of diseases that affect the nervous system such as Parkinson’s disease [5] , [7] , [8] , [9] , [10] . The worm, C. elegans , and the fruit fly, Drosophila melanogaster , have served as animal models for characterizing proprioception. Both of these organisms display highly stereotypic locomotion [11] , [12] , [13] , [14] , [15] , which has facilitated the identification of neurons and ion channels that function in proprioception [14] , [15] , [16] , [17] , [18] . In flies, proprioceptive neurons are located in specialized sensory structures—mechanosensory bristles, campaniform sensilla, and chordotonal organs [19] . Several invertebrate members of the transient receptor potential (TRP) family of cation channels localize to proprioceptive cells and contribute to sensing bodily movements during locomotion. These include the C. elegans and Drosophila TRPN channels, TRP-4 and NOMPC, respectively, which are required for worms and fly larvae to make gross postural changes during locomotion [14] , [17] , [20] . Most nompC mutant animals die during the pupal stage [20] , [21] . The few mutant animals that survive to adulthood exhibit severe locomotion defects and uncoordinated movement of body parts, indicative of defects in gross motor control [17] . Mutations disrupting the Drosophila TRPV channels, Inactive (Iav) and Nanchung (Nan) also result in severe locomotor defects [11] , [22] , [23] , [24] . A key question is whether ion channels exist that specifically function in fine motor control. In flies, a defect in fine motor control would not eliminate behaviours that rely principally on gross movements of the body and appendages, such as negative geotaxis, or crossing small gaps. However, loss of fine motor control would be expected to impair performance when the flies are faced with highly challenging tasks, such as traversing wide gaps, which rely on coordinating a repertoire of fine movements, including subtle changes in body angles and leg positions [11] , [12] . The Drosophila genome encodes 13 TRPs, 12 of which have been subjected to genetic analyses [16] , [25] . The recurring theme is that these channels are essential for sensory physiology. However, the function of one Drosophila TRP channel, TRPγ, is not known. TRPγ is a TRPC channel [26] , and is most related to the founding TRP channel [27] . In this study we demonstrate that TRPγ is localized to neurons and glia that comprise the femoral chordotonal organs (FCOs). We generated trpγ null mutant flies and found that they were distinct from the nan and iav mutants in that they displayed much greater levels of negative geotaxis and were proficient in crossing small gaps. However, once the gaps became challenging but were still surmountable for most wild-type flies, the trpγ mutants were unable to make the fine postural adaptations required for negotiating these gaps. Thus, this phenotype sharply contrasted with the loss of other TRP channels that impact on proprioception, as TRPγ was uniquely required to promote this highly coordinated motor control. These data demonstrate that fine motor control is not mediated exclusively through the same repertoire of cation channels that function in gross motor control. Expression of the trpγ reporter in proprioceptive organs To obtain clues as to the roles of trpγ , we generated a gene reporter to examine its expression pattern. We used homologous recombination [28] to insert the yeast GAL4 gene at the site of the ATG. To simultaneously generate a mutant allele, we deleted 547 base pairs extending 3′ from the start codon with the GAL4 gene ( trpγ G4 ; Fig. 1a,b ). Using trpγ G4 /+ in conjunction with UAS-DsRed , we found that the trpγ reporter was expressed prominently in FCOs ( Fig. 1c,d ), which are responsible for sensing stretch and the position of the fly legs [29] . The reporter also labelled neurons in macrochaetes (mechanosensory bristles) [20] on the dorsal thorax and legs ( Fig. 1e,f ). 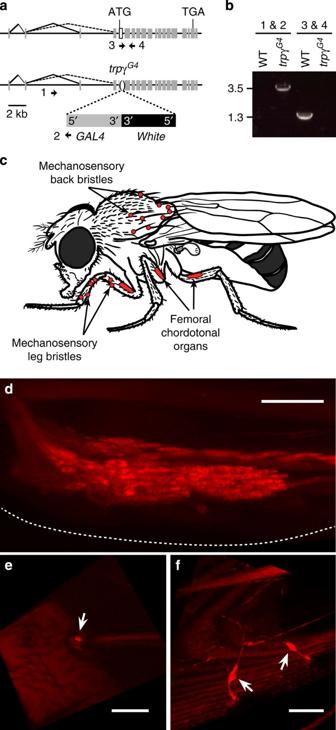Figure 1: Expression of thetrpγreporter in mechanosensitive and proprioceptive organs. (a) Schematic of thetrpγgene andtrpγG4knockout generated by ends-out homologous recombination28. (b) PCR amplification of genomic DNA to identify flies with thetrpγG4mutation. The positions of the primer pairs that were used are indicated ina. The upper and lower tick marks to the left represent the positions of the 3.5 and 1.3-kb markers. (c) Cartoon depicting the location of mechanosensitive sensilla and proprioceptive organs distributed on the fly. Sites of prominenttrpγreporter expression are labelled in red. (d–f) Expression of thetrpγG4reporter (trpγG4/+;UAS-dsRed).Scale bars, 20 μm. (d) FCO in a foreleg. (e) The white arrow indicates a neuron innervating a macrochaete in the dorsal thorax. (f) The white arrows indicate neurons innervating large mechanosensory bristles of the femoral segment of the foreleg. Figure 1: Expression of the trpγ reporter in mechanosensitive and proprioceptive organs. ( a ) Schematic of the trpγ gene and trpγ G4 knockout generated by ends-out homologous recombination [28] . ( b ) PCR amplification of genomic DNA to identify flies with the trpγ G4 mutation. The positions of the primer pairs that were used are indicated in a . The upper and lower tick marks to the left represent the positions of the 3.5 and 1.3-kb markers. ( c ) Cartoon depicting the location of mechanosensitive sensilla and proprioceptive organs distributed on the fly. Sites of prominent trpγ reporter expression are labelled in red. ( d – f ) Expression of the trpγ G4 reporter ( trpγ G4 /+; UAS-dsRed). Scale bars, 20 μm. ( d ) FCO in a foreleg. ( e ) The white arrow indicates a neuron innervating a macrochaete in the dorsal thorax. ( f ) The white arrows indicate neurons innervating large mechanosensory bristles of the femoral segment of the foreleg. Full size image TRPγ was required for the rapid righting reflex The expression of the trpγ reporter in proprioceptive organs raised the possibility that TRPγ was required for coordination or locomotor activity. To examine the role of TRPγ we characterized trpγ G4 animals, as well as a second mutant allele, trpγ 1 , which we generated by homologous recombination ( Supplementary Fig. 1a,b ). The trpγ 1 mutation removed 180 base pairs that encoded the carboxyl-terminal portion of the sixth transmembrane domain as well as the highly conserved TRP box (EWKFAR) [30] . Both trpγ 1 and trpγ G4 were homozygous viable and fertile. To assay overall locomotor activity, we used an actometer ( Drosophila Activity Monitoring System) and found that the mutant flies showed a decrease in overall activity ( Supplementary Fig. 2a ). Both trpγ 1 and trpγ G4 mutant flies also displayed a small but significant negative geotaxis defect, which we assayed by gently tapping down the flies in a graduated cylinder ( Supplementary Fig. 2b ). However, in contrast to the severe reduction in climbing indexes exhibited by flies missing either of the TRPV channels, Nan ( nan 36a ) and Iav ( iav 1 ; originally called hypo B ) [22] , [23] , the trpγ mutant flies showed only mild impairments in this behaviour ( Supplementary Fig. 2b ). Wild-type flies have a rapid righting reflex, which depends on using alternating legs to push against the ground, thereby enabling them to turn over. Because the speed of this reflex requires coordinated movements of the legs, we wondered whether the turnover behaviour was impaired in the mutant animals. After taping down flies in a cylinder, wild-type flies righted themselves in slightly more than 1 second (1.19±0.24 s, mean±s.e.m. ; Fig. 2a ; Supplementary Fig. 2c and Supplementary Movie 1 ). In contrast, trpγ 1 and trpγ G4 animals required four times longer to complete the righting reflex (4.76±2.39 and 3.72±1.81 s, respectively; Fig. 2a ; Supplementary Fig. 2c ). This delay in righting did not appear to be due to defects in sensing the supine position, as the mutant flies were actively engaged in righting attempts immediately after the tap down, similar to the wild type. We rescued this phenotype with either a genomic transgene ( gtrpγ ) or with a UAS-trpγ transgene, using the GAL4 inserted into trpγ G4 (1.11±0.45 and 1.76±0.68 s, respectively; Fig. 2a ). 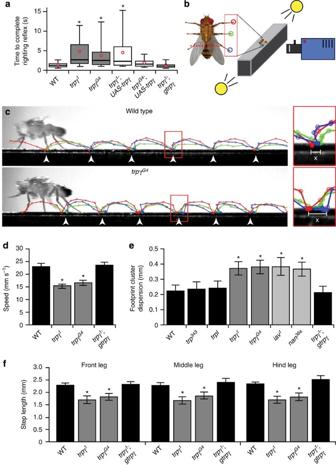Figure 2: Comparison of wild-type andtrpγrighting reflex and leg coordination during walking. (a) Quantification of the righting reflex. In each box plot the solid black bar represents the median value and open red circle represents the mean. The boxes denote the 25 and 75% quantiles of the distribution. The whiskers represent 5 and 95% quantiles. Wild-type, WT. Non-parametric Mann–WhitneyU-test,n≥100. *P≤0.05. (b) Schematic of the catwalk behavioural set-up. To track the movements of the leg tips on one side of the body, we positioned a high-resolution, high-frame rate camera orthogonally at the level of the catwalk: front (red), middle (green), and hind (blue). The wings were clipped (red dashed line) to prevent the animal from flying. We recorded at 250 fps. (c) Representative crossings of wild-type andtrpγG4flies showing footprint clustering on the catwalk. Footprint cluster dispersions (X, red inset boxes enlarged in the right panel) were measured as the width of each cluster using the initial contact point on the platform for each leg. (d) Average walking speed of flies across the catwalk. (e) Footprint cluster dispersion during walking. (f) Quantification of step length for the front, middle and hind legs during walking. Mean±s.e.m.,n≥5. Analysis of variance with Dunnet’spost hocanalysis. *P≤0.05. Figure 2: Comparison of wild-type and trpγ righting reflex and leg coordination during walking. ( a ) Quantification of the righting reflex. In each box plot the solid black bar represents the median value and open red circle represents the mean. The boxes denote the 25 and 75% quantiles of the distribution. The whiskers represent 5 and 95% quantiles. Wild-type, WT. Non-parametric Mann–Whitney U -test, n ≥100. * P ≤0.05. ( b ) Schematic of the catwalk behavioural set-up. To track the movements of the leg tips on one side of the body, we positioned a high-resolution, high-frame rate camera orthogonally at the level of the catwalk: front (red), middle (green), and hind (blue). The wings were clipped (red dashed line) to prevent the animal from flying. We recorded at 250 fps. ( c ) Representative crossings of wild-type and trpγ G4 flies showing footprint clustering on the catwalk. Footprint cluster dispersions (X, red inset boxes enlarged in the right panel) were measured as the width of each cluster using the initial contact point on the platform for each leg. ( d ) Average walking speed of flies across the catwalk. ( e ) Footprint cluster dispersion during walking. ( f ) Quantification of step length for the front, middle and hind legs during walking. Mean±s.e.m., n ≥5. Analysis of variance with Dunnet’s post hoc analysis. * P ≤0.05. Full size image Loss of trpγ impaired fine leg coordination during walking The defect in the righting reflex suggested that leg movement coordination might be compromised in the trpγ mutants. To assess this question quantitatively, we performed a video analysis of flies walking over a catwalk. We mounted the camera orthogonally to the catwalk at the level of the walking surface, and recorded at an increased speed (200–250 frames s −1 ) as the flies traversed the platform ( Fig. 2b ). We tracked the movements of the three legs facing the camera or the set facing away. From this perspective, the leg movements of wild-type animals were highly coordinated such that all three legs contacted the catwalk on nearly the same points ( Fig. 2c and Supplementary Movie 2 ), due to the flies alternating tripod gait [11] , [13] . From these leg tracks, we measured the walking speed, the inter-step distances for the front, middle and hind legs, as well as the dispersion of the footprint clusters ( Fig. 2d–f ). We found that loss of trpγ reduced the speed and precision of movements during walking ( Supplementary Movie 3 ). The trpγ mutant animals showed a 28–33% decrease in forward walking speed (wild type, 22.7±1.5 mm s −1 , mean±s.e.m. ; trpγ 1 , 15.2±0.2 mm s −1 ; trpγ G4 , 16.3±0.4 mm s −1 ; Fig. 2d ) accompanied by a 19–25% shorter average step length (wild-type, 2.28±0.08 mm, mean±s.e.m. ; trpγ 1 , 1.70±0.15 mm; trpγ G4 , 1.84±0.14 mm; Fig. 2f ). Of greatest significance from the perspective of coordination, the footprint cluster dispersions of trpγ 1 and trpγ G4 were increased ∼ 60% (wild-type, 0.23±0.04 mm, mean±s.e.m. ; trpγ 1 , 0.39±0.07 mm; trpγ G4 , 0.36±0.05 mm; Fig. 2e ). The iav 1 and nan 36a mutants displayed similar footprint cluster dispersion deficits ( iav 1 , 0.39±0.08 mm; nan 36a , 0.36±0.06 mm; Fig. 2e ). We did not analyse nompC mutants since too few of these animals survived to adulthood. Introduction of the wild-type trpγ genomic transgene ( gtrpγ ) rescued the walking defects displayed by trpγ mutants ( Fig. 2d–f ). trpγ mutants showed defects in traversing large gaps To further evaluate leg coordination in trpγ 1 and trpγ G4 , we increased the difficulty of the locomotor task by adding gaps of varying widths to the catwalk. The number of approaches per attempt increased with the gap width ( Fig. 3a,b ). If the gaps were relatively short (2.5 mm), most approaches by wild-type flies were followed by an attempt at a gap crossing (1.3±0.4 approaches per attempt, mean±s.e.m. ; Fig. 3b ). If the gap width was increased to 4.0 mm, then the number of approaches per attempt nearly doubled (2.4±0.1 approaches per attempt; Fig. 3b ). 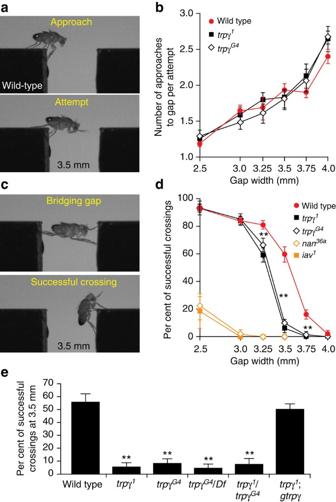Figure 3: Assaying wild-type andtrpγgap crossing at various gap widths. We recorded videos at 250 fps. (a) Still frames from the video showing a male wild-type fly during a gap crossing at 3.5 mm. We defined the approach posture (upper panel) as a pause at the gap with three legs on the starting wall. We defined an attempt (lower panel), as repeated LOH motions/strokes towards the opposite side of the gap. (b) Number of approaches per attempt at crossing, as a function of the gap width. (c) Still frames from a video showing a wild-type male fly successfully crossing a 3.5 mm gap. The fly bridged the gap with its front and hind legs (upper panel). After gripping the opposite side with its front legs, the fly released its hind legs, which allowed its body to swing across the gap (lower panel). (d) Per cent of successful crossings. The percentages were based on 10 attempts per fly at different gap widths. Analysis of variance (ANOVA) with Dunnet’spost hocanalysis,n≥10, **P≤0.01. (e) Quantification of gap crossing success at 3.5 mm for the animals with the indicated genotypes. ANOVA with Dunnet’spost hocanalysis.n≥10, **P≤0.01. Figure 3: Assaying wild-type and trpγ gap crossing at various gap widths. We recorded videos at 250 fps. ( a ) Still frames from the video showing a male wild-type fly during a gap crossing at 3.5 mm. We defined the approach posture (upper panel) as a pause at the gap with three legs on the starting wall. We defined an attempt (lower panel), as repeated LOH motions/strokes towards the opposite side of the gap. ( b ) Number of approaches per attempt at crossing, as a function of the gap width. ( c ) Still frames from a video showing a wild-type male fly successfully crossing a 3.5 mm gap. The fly bridged the gap with its front and hind legs (upper panel). After gripping the opposite side with its front legs, the fly released its hind legs, which allowed its body to swing across the gap (lower panel). ( d ) Per cent of successful crossings. The percentages were based on 10 attempts per fly at different gap widths. Analysis of variance (ANOVA) with Dunnet’s post hoc analysis, n ≥10, ** P ≤0.01. ( e ) Quantification of gap crossing success at 3.5 mm for the animals with the indicated genotypes. ANOVA with Dunnet’s post hoc analysis. n ≥10, ** P ≤0.01. Full size image The increase in approaches per attempt was inversely proportional to success of the the wild-type flies to traverse the gap. At a gap width of 2.5 mm, 93±2.6% of the attempts (mean±s.e.m.) were successful ( Fig. 3c,d ). A majority of crossing attempts were still successful at 3.5 mm (59.2±5.3%; Fig. 3c–e ) a gap width ∼ 1.5 times the flies’ average body length of 2.26±0.04 mm (mean±s.e.m., Fig. 3a,b and Supplementary Table 1 ). A minority of crossing attempts was successful at the 3.75 mm gap (16.0±3.4%; Fig. 3d ), and very few flies were able to surmount a 4.0 mm divide (2.0±1.3%; Fig. 3d ). The trpγ 1 and trpγ G4 animals initiated gap crossing with a frequency similar to wild type ( Fig. 3b ), but were impaired in traversing larger gaps ( Fig. 3d ). At distances of ≤3.0 mm, trpγ mutant animals were equally successful at negotiating gaps as wild-type flies ( Fig. 3d ). However, their success was reduced significantly as the sizes of the openings increased. The differences between wild-type and the mutants were most pronounced at the 3.5-mm gap width. Wild-type animals crossed this gap more than half of the time. However, the 3.5-mm opening was nearly insurmountable for the trpγ mutants ( trpγ 1 , 6.0±3.4%; trpγ G4 , 8.4±2.7%; Fig. 3d,e ). This ineffectiveness was not due to a shorter body length ( trpγ 1 , 2.29±0.02 mm; trpγ G4 , 2.17±0.03 mm; Fig. 4a,b and Supplementary Table 1 ). The gap-crossing impairment reflected a requirement for the trpγ gene, since we observed the same phenotype in both mutant alleles, in trans-heterozygous flies, and when we placed the trpγ 1 mutation in trans with a deficiency uncovering the mutation ( Fig. 3e ). We restored normal crossing ability with a wild-type gtrpγ genomic transgene ( trpγ 1 ; gtrpγ 50.5±3.8%; Fig. 3e ). The trpγ phenotype was distinct from iav 1 and nan 36a mutants, which failed in their attempts at surmounting much shorter gap distances ( Fig. 3d ). 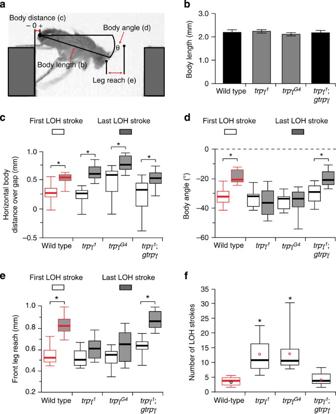Figure 4: Abilities oftrpγmutants to make the fine postural adaptions necessary to fully extend their reach during gap crossing. (a) Illustration of the different postural metrics extracted from gap crossing videos recorded at 200 fps. (b) Quantification of body lengths. Mean±s.e.m.,n≥10. Lack of statistical significance was determined by analysis of variance. (c) Quantification of the changes in horizontal body position over the gap from the first LOH stroke (open boxes) to the last LOH stroke (grey filled boxes). (d) Quantification of the changes in body angle towards horizontal from first LOH to last LOH. (e) Quantification of the changes in front leg reach from first LOH to last LOH. (f) Quantification of the total number of LOH strokes performed by each fly during a crossing attempt at 3.5 mm. For each box plot inc–f, the solid bar represents the median value, the box denotes the 25 and 75% quantiles of the distribution, and the whiskers represent 5 and 95% quantiles. Forc–e, the statistical significances were determined by non-parametric Wilcoxon signed-rank tests,n≥10, *P≤0.05. Forf, the open circles represent the mean value. Statistical significances were determined by non-parametric Mann–WhitneyU-tests.n≥10, *P≤0.05. Figure 4: Abilities of trpγ mutants to make the fine postural adaptions necessary to fully extend their reach during gap crossing. ( a ) Illustration of the different postural metrics extracted from gap crossing videos recorded at 200 fps. ( b ) Quantification of body lengths. Mean±s.e.m., n ≥10. Lack of statistical significance was determined by analysis of variance. ( c ) Quantification of the changes in horizontal body position over the gap from the first LOH stroke (open boxes) to the last LOH stroke (grey filled boxes). ( d ) Quantification of the changes in body angle towards horizontal from first LOH to last LOH. ( e ) Quantification of the changes in front leg reach from first LOH to last LOH. ( f ) Quantification of the total number of LOH strokes performed by each fly during a crossing attempt at 3.5 mm. For each box plot in c – f , the solid bar represents the median value, the box denotes the 25 and 75% quantiles of the distribution, and the whiskers represent 5 and 95% quantiles. For c – e , the statistical significances were determined by non-parametric Wilcoxon signed-rank tests, n ≥10, * P ≤0.05. For f , the open circles represent the mean value. Statistical significances were determined by non-parametric Mann–Whitney U -tests. n ≥10, * P ≤0.05. Full size image Impairments in postural adaptations to fully extend reach Gap crossing is a highly stereotyped behaviour that flies perform by making progressive postural adjustments in their horizontal body distance, body angle and front leg reach ( Fig. 4a and Supplementary Movie 4 ) [12] . To assay the horizontal body distance and postural adaptations in body angle, we tracked both the head and posterior positions of the flies during crossings over a 3.5-mm gap. As soon as wild-type flies extended their bodies over a gap to attempt a crossing, they began to perform leg over head (LOH) strokes ( Fig. 4a and Supplementary Movie 4 ). With each subsequent LOH stroke, the flies adjusted their posture aiming to maximize their reach across the gap. We compared the body positions and angles at the initiation of each crossing (first LOH stroke) and at the end of each crossing, just before the front legs contacted the opposite side, or when the flies gave up and turned back (last LOH stroke). Wild-type flies increased their horizontal body positions by 0.23±0.05 mm (mean±s.e.m., Fig. 4c ) and flattened their body angles towards horizontal by 13.6±2.3° (mean±s.e.m., Fig. 4d ). To assay the front leg reach postural adaptation, we tracked the positions of the flies’ front legs relative to the head during crossings. Wild-type flies extended their front legs during gap crossing, and improved their reach by 0.26±0.04 mm (mean±s.e.m., Fig. 4e ). We found that the trpγ mutant animals were unable to optimally perform postural adjustments while attempting to cross a 3.5-mm gap ( Supplementary Movie 5 ). The trpγ 1 and trpγ G4 flies were able to increase their horizontal body distances over the gap (0.42±0.06 and 0.39±0.11 mm, respectively; Fig. 4c ). However, in contrast to the wild type, the body angles of the trpγ mutants remained near their starting angles and did not increase throughout their crossing attempts ( trpγ 1 , −1.9±2.8° and trpγ G4 , −1.5±3.5°; Fig. 4d ). In addition, the trpγ mutant flies did not fully extend their front legs ( trpγ 1 , 0.09±0.03 mm; trpγ G4 , 0.13±0.06 mm; Fig. 4e ). After we introduced a wild-type trpγ transgene ( gtrpγ ), in the trpγ 1 background, all of the postural adjustments were similar to the wild type (body distance, 0.31±0.08 mm; body angle, 10.6±1.5°; front leg reach, 0.23±0.04 mm; Fig. 4c–e ). With each LOH stroke, wild-type flies update their body posture as they attempt to bridge a gap. The total number of LOH strokes is tightly regulated in wild-type flies as this is thought to reduce the expenditure of energy during attempts to traverse insurmountable gaps [12] . Wild-type flies performed 3.6±0.4 LOH strokes during a 3.5 mm crossing (mean±s.e.m., Fig. 4f ). The trpγ 1 and trpγ G4 mutants performed 3.4 to 4.0 times more LOH strokes, and the variation in number was much greater than was typical of wild-type flies (12.2±2.0 and 14.5±2.5 strokes, respectively; Fig. 4f ). Some of the trpγ mutant flies produced strikingly large numbers of LOH strokes such that the maximum number was up to 10 times greater than the wild type ( Fig. 4f ). Introduction of gtrpγ in trpγ 1 animals restored a level of LOH strokes that was similar to wild type (4.82±0.72 strokes; Fig. 4f ). Localization of TRPγ in the femoral chordotonal organs The FCO is located in the proximal part of each femoral leg segment ( Fig. 5a ), and is comprised of three large groups of aligned scolopidia ( Fig. 5b ). Each group contains between 10 to 35 scolopidia ( Fig. 5c ) [31] . 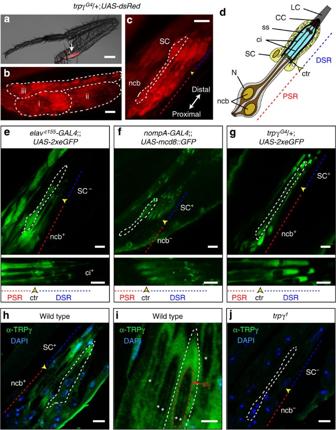Figure 5: TRPγ localizes to neurons and scolopale cells of femoral chordotonal organs. (a) ThetrpγG4reporter droveUAS-dsRedexpression in the FCO of the forelegs (white arrow). Scale bar, 100 μm. (b)trpγG4staining of the three bundles/groups of aligned scolopidia, i, ii and iii that comprise the FCO (dashed lines). Scale bar, 10 μm. (c) Reconstruction oftrpγG4FCO staining revealing the structure of multiple, aligned scolopidia. Neuronal cell bodies (ncb) and scolopale cells (SC) are situated in the PSR and the DSR, respectively. Scale bar, 10 μm. (d) Schematic of an individual scolopidia showing the neurons (N), neuron cell bodies (ncb), cilia (ci), cap cell (CC), ligament cell (LC), scolopale cell (SC) and scolopale space (ss). Ciliary transition root (ctr, yellow arrow) demarcates the PSR (red dashed line) and DSR (blue dashed line). (e–j) Staining of FCO scolopidia bundles. White dashed line outlines single scolopidia units. Scale bars, 5 μm. (e) Pan-neuronalelavc155-Gal4staining revealed fluorescence in neuron cell bodies (ncb+) and in the scolopale cell layer, but not in scolopale cells (SC–). Staining of thin-paired cilia (ci+) was seen in the DSR. The distal ends of the scolopidia are enlarged for detail (bottom panel). (f) Scolopale cell-specificnompA-Gal4staining revealed fluorescence only in the scolopale cells (SC+) and not in the neuron cell bodies (ncb–). Neither axonal nor ciliary signal was detected usingnompA-Gal4(bottom panel). (g) ThetrpγG4reporter stained both neuronal cell bodies (ncb+) and scolopale cells (SC+). Staining of the scolopale cells obscured the sensory cilia (bottom panel). (h) Longitudinal section of wild-type FCO immunostained with α–TRPγ and counterstained with DAPI. Antibodies strongly labelled the distal ends of the scolopale cells (SC+), and more diffusely labelled neuron cell bodies (ncb+). (i) Enlarged view of the DSR showing multiple scolopale spaces (ss, red dashed line). Within the ss, α–TRPγ stained cilia, but labelling of such thin processes was weak (white asterisks, at the proximal end of each cilia). (j) Longitudinal section oftrpγ1FCO immunostained with α–TRPγ and counterstained with DAPI. Figure 5: TRPγ localizes to neurons and scolopale cells of femoral chordotonal organs. ( a ) The trpγ G4 reporter drove UAS-dsRed expression in the FCO of the forelegs (white arrow). Scale bar, 100 μm. ( b ) trpγ G4 staining of the three bundles/groups of aligned scolopidia, i, ii and iii that comprise the FCO (dashed lines). Scale bar, 10 μm. ( c ) Reconstruction of trpγ G4 FCO staining revealing the structure of multiple, aligned scolopidia. Neuronal cell bodies (ncb) and scolopale cells (SC) are situated in the PSR and the DSR, respectively. Scale bar, 10 μm. ( d ) Schematic of an individual scolopidia showing the neurons (N), neuron cell bodies (ncb), cilia (ci), cap cell (CC), ligament cell (LC), scolopale cell (SC) and scolopale space (ss). Ciliary transition root (ctr, yellow arrow) demarcates the PSR (red dashed line) and DSR (blue dashed line). ( e – j ) Staining of FCO scolopidia bundles. White dashed line outlines single scolopidia units. Scale bars, 5 μm. ( e ) Pan-neuronal elav c155 -Gal4 staining revealed fluorescence in neuron cell bodies (ncb + ) and in the scolopale cell layer, but not in scolopale cells (SC – ). Staining of thin-paired cilia (ci + ) was seen in the DSR. The distal ends of the scolopidia are enlarged for detail (bottom panel). ( f ) Scolopale cell-specific nompA-Gal4 staining revealed fluorescence only in the scolopale cells (SC + ) and not in the neuron cell bodies (ncb – ). Neither axonal nor ciliary signal was detected using nompA-Gal4 (bottom panel). ( g ) The trpγ G4 reporter stained both neuronal cell bodies (ncb + ) and scolopale cells (SC + ). Staining of the scolopale cells obscured the sensory cilia (bottom panel). ( h ) Longitudinal section of wild-type FCO immunostained with α–TRPγ and counterstained with DAPI. Antibodies strongly labelled the distal ends of the scolopale cells (SC + ), and more diffusely labelled neuron cell bodies (ncb + ). ( i ) Enlarged view of the DSR showing multiple scolopale spaces (ss, red dashed line). Within the ss, α–TRPγ stained cilia, but labelling of such thin processes was weak (white asterisks, at the proximal end of each cilia). ( j ) Longitudinal section of trpγ 1 FCO immunostained with α–TRPγ and counterstained with DAPI. Full size image A scolopidium is the fundamental mechanosensitive unit of the insect chordotonal organ and consists of four cell types: (1) two bipolar neurons (N), (2) one glial cell (scolopale cell; SC), (3) one cap cell (CC) and (4) one ligament cell (LC; Fig. 5d ) [19] . The dendrites of the bipolar neurons have two distinct regions demarcated by a ciliary transition root (ctr, yellow arrow; Fig. 5d ). In the proximal scolopidial region (PSR), the dendrites are larger in diameter than in the distal scolopidial region (DSR; red and blue dashed lines, respectively; Fig. 5d ). The scolopale cell encloses a wide extracellular space (scolopidial space; ss). The thin sensory cilia (ci), which comprise the distal region of the dendrites, extend through the scolopidial space and terminate at the cap cell. The cap cell mechanically couples the scolopidium to either the epicuticular surface or femoral muscle membranes via a ligament cell ( Fig. 5d ). The distinctive morphologies and positions of the cells within a scolopidium allowed us to identify the cell types labelled by the trpγ reporters. The neuronal-specific marker, elav-GAL4 , labelled the neuronal cell bodies (ncb+) in the PSR (red dashed line; Fig. 5e ). This reporter also stained the ciliary transition roots (ctr, yellow arrow) and the sensory cilia (ci+, blue dashed line), but not the scolopale cells (SC−; Fig. 5e lower panel). The labelling of the sensory cilia was weak due to the narrow diameter of these dendrites. To specifically mark the scolopale cells, we used the nompA - GAL4 (refs 32 , 33 ; Fig. 5f ; SC+, blue dashed line). The SC+ staining was considerably wider in diameter than either the proximal or distal dendritic signals, consistent with the morphology of scolopale cells. We found that the trpγ reporter ( trpγ G4 /+) stained both neurons and glia (scolopale cells) in the FCO. Consistent with neuronal expression, the trpγ GAL4 stained the neuronal cell bodies (ncb+), and the proximal dendritic projections in the PSR (red dashed line; Fig. 5g ). The reporter also marked the ciliary transition roots (ctr, yellow arrow) and cells in the DSR (blue dashed line; Fig. 5g ). The morphology of these distal cells was consistent with expression in scolopale cells (SC+; Fig. 5g , upper and lower panel). To confirm that the trpγ reporter reflected the bona fide expression pattern, and to determine the subcellular localization of the TRPγ protein, we generated TRPγ antibodies (α–TRPγ). The antibody accessibility was poor in whole-mount leg samples and standard fixation methods followed by frozen or resin embedded sectioning resulted in damaged FCO morphology. Therefore, to better preserve the FCO ultrastructure, we subjected whole legs to high-pressure freezing followed by low-temperature fixation and embedding though automated freeze substitution [34] . We immunostained sections, and found that the α–TRPγ antibodies labelled the proximal dendrites and neuronal cell bodies (ncb+) in the PSR (red dashed line) and the scolopale cells (SC+) surrounding the scolopidial spaces in the DSR (blue dashed line; Fig. 5h ). Labelling was strongest towards the distal ends of the scolopale cells, while the signal in the neuron cell bodies was more diffuse (ncb+). We also detected weak α–TRPγ signals in the extremely thin sensory cilia in the scolopidial spaces (white asterisks, placed at proximal end of visible cilia signal; Fig. 5i ). Neither of the two neuronal-specific antibodies (anti-ELAV or anti-22C10) stained these sections, precluding double-labelling experiments. Nevertheless, the α–TRPγ signal appeared to be specific since we did not detect staining in the trpγ 1 mutant ( Fig. 5j ). Loss of TRPγ disrupted the resistance reflex To assess the functional consequences due to the loss of TRPγ, we performed extracellular myogram (EMG) recordings and measured the resistance reflex in muscle cells that depended on functional neurons in FCOs [35] , [36] , [37] , [38] . We placed a sharp borosilicate electrode under the cuticle of the femur and recorded excitatory responses from the tibial extensor muscles in response to rhythmic movement of the tibia about the femoral joint. A 2-Hz movement of the wild-type tibia elicited robust firing of the slow extensor motor neurons ( Fig. 6a,c ; 107.2±11.5 spikes per 360° cycle of movement, mean±s.e.m.). We found that these motor neurons were silent in the absence of flexion. However, trpγ mutant animals displayed ∼ 40–58% reductions in the frequencies of action potentials in response to tibia deflections ( Fig. 6b,c ; trpγ 1 , 64.8±8.6 spikes per cycle; trpγ G4 , 64.4±7.5 spikes per cycle; trpγ 1 / trpγ G4 , 45.8±8.3 spikes per cycle). While the frequencies of action potentials were decreased, the mutant animals retained synchronous firing patterns. We restored a wild-type level of action potentials with a genomic transgene ( Fig. 6c ; trpγ 1 ;gtrpγ ; 105.0±13.6 spikes per cycle), or by expressing a trpγ transgene ( UAS-trpγ ) under control of the trpγ promoter ( GAL4 knocked into trpγ locus; Fig. 6c ; trpγ G4 /trpγ 1 ,UAS-trpγ ; 107.2±13.0 spikes per cycle). 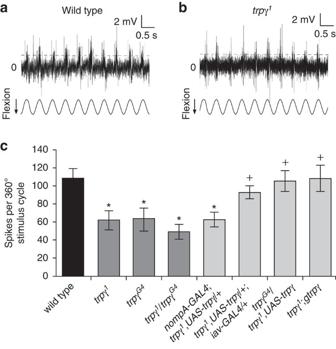Figure 6: Assaying tibial extensor muscle activity by EMG recordings. (aandb) Representative EMG recordings of tibial extensor muscle activity in response to tibial flexion at 2 Hz. The grey dashed line represents a spike detector threshold 10% above the 1 s mean noise before stimulation. (c) Quantification of the change in the number of spikes elicited per 360° of flexion for flies of different genotypes. Mean±s.e.m.,n≥5. Analysis of variance with Dunnet’spost hocanalysis. *P≤0.05 with wild type as control group.+P≤0.05 withtrpγ1as the control group. Figure 6: Assaying tibial extensor muscle activity by EMG recordings. ( a and b ) Representative EMG recordings of tibial extensor muscle activity in response to tibial flexion at 2 Hz. The grey dashed line represents a spike detector threshold 10% above the 1 s mean noise before stimulation. ( c ) Quantification of the change in the number of spikes elicited per 360° of flexion for flies of different genotypes. Mean±s.e.m., n ≥5. Analysis of variance with Dunnet’s post hoc analysis. * P ≤0.05 with wild type as control group. + P ≤0.05 with trpγ 1 as the control group. Full size image Cell-type requirement for trpγ in chordotonal organs To determine the cell type-specific requirement for TRPγ for the mechanically evoked response, we recorded EMGs from trpγ null animals after restoring trpγ expression ( UAS-trpγ ) only in chordotonal neurons ( iav-GAL4 ) or in scolopale cells ( nompA-GAL4 ). We found that the expression of trpγ in chordotonal neurons but not scolopale cells rescued the trpγ EMG phenotype ( Fig. 6c ; 91.6±7.6 spikes per cycle and 63.8±6.2 spikes per cycle, respectively). To investigate the cellular requirement for TRPγ for successful gap crossing, we performed RNA interference (RNAi) knockdown and UAS-trpγ rescue experiments. We assayed for proficiency at traversing 3.5 mm gaps. The UAS - trpγ RNAi was effective, since we phenocopied the gap-crossing deficit using the trpγ G4 (compare trpγ G4 /+ with and without the UAS - trpγ RNAi; Fig. 7a ). We recapitulated the trpγ mutant phenotype using all three neuronal drivers tested: elav-GAL4 , nanchung ( nan ) -GAL4 or inactive ( iav ) -GAL4 ( Fig. 7a ). Knockdown of UAS - trpγ in scolopale cells using the nompA-Gal4 impaired gap crossing, through not to the same extent as the neuronal GAL4 drivers ( Fig. 7a ). Knockdown of trpγ with a cap cell-specific GAL4 , pyrexia (pyx)-GAL4 (ref. 39 ), did not affect gap crossing ( Fig. 7a ). We also tested the atonal (ato)-GAL4 , which is expressed in both neurons and scolopale cells of the chordotonal Johnston’s organ [33] . However, the ato-GAL4 did not cause any effect in the RNAi experiments ( Fig. 7a ), or drive detectable UAS-GFP expression in the FCO. 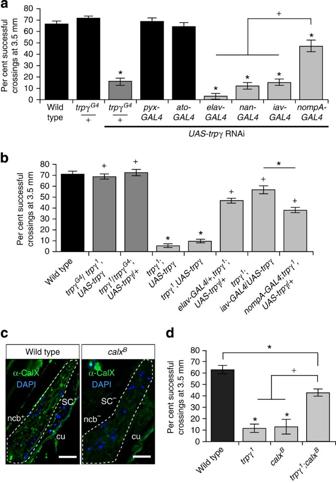Figure 7: TRPγ dependent Ca2+influx is required in neurons and scolopale cells for effective gap crossing. (a) Percentage of animals that were successful at crossing a 3.5 mm gap after knocking downtrpγ(UAS-trpγRNAi) with the indicatedGAL4drivers. Mean±s.e.m.,n≥30. Analysis of variance (ANOVA) with Dunnet’spost hocanalysis. *P≤0.05 with wild type as the control group. (b) Gap-crossing success (3.5 mm gap) oftrpγ1flies that expressedUAS-trpγunder the control of a variety ofGal4drivers. Data are presented as mean±s.e.m.,n≥30. ANOVA with Dunnet’spost hocanalysis. *P≤0.05 with wild type as the control group.+P≤0.05 withUAS-trpγon the second or third chromosome in atrpγ1mutant background as the control group. (c) Longitudinal section through a wild type andcalxBFCO immunostained with α–CalX and counterstained with DAPI. The antibodies labelled the scolopale cells (SC+), and neuron cell bodies (ncb+) in wild-type sections only. Nonspecific staining of the cuticle (cu) occurred in both the wild-type and mutant sections. Scale bars, 10 μm. (d) Gap-crossing success (3.5 mm gap) oftrpγ1, calxB, and thetrpγ1;calxBdouble mutant. Data are presented as mean±s.e.m.,n≥10. ANOVA with Tukey’spost hocanalysis. *P≤0.05. Figure 7: TRPγ dependent Ca 2+ influx is required in neurons and scolopale cells for effective gap crossing. ( a ) Percentage of animals that were successful at crossing a 3.5 mm gap after knocking down trpγ ( UAS-trpγ RNAi) with the indicated GAL4 drivers. Mean±s.e.m., n ≥30. Analysis of variance (ANOVA) with Dunnet’s post hoc analysis. * P ≤0.05 with wild type as the control group. ( b ) Gap-crossing success (3.5 mm gap) of trpγ 1 flies that expressed UAS-trpγ under the control of a variety of Gal4 drivers. Data are presented as mean±s.e.m., n ≥30. ANOVA with Dunnet’s post hoc analysis. * P ≤0.05 with wild type as the control group. + P ≤0.05 with UAS-trpγ on the second or third chromosome in a trpγ 1 mutant background as the control group. ( c ) Longitudinal section through a wild type and calx B FCO immunostained with α–CalX and counterstained with DAPI. The antibodies labelled the scolopale cells (SC + ), and neuron cell bodies (ncb + ) in wild-type sections only. Nonspecific staining of the cuticle (cu) occurred in both the wild-type and mutant sections. Scale bars, 10 μm. ( d ) Gap-crossing success (3.5 mm gap) of trpγ 1 , calx B , and the trpγ 1 ; calx B double mutant. Data are presented as mean±s.e.m., n ≥10. ANOVA with Tukey’s post hoc analysis. * P ≤0.05. Full size image We also tested for rescue of the trpγ gap crossing defects with a wild-type trpγ transgene. Introduction of the UAS-trpγ transgene in trpγ G4 / trpγ 1 flies fully rescued the mutant phenotype ( Fig. 7b ). The rescue required the trpγ G4 driver since the UAS-trpγ transgenes did not restore gap-crossing performance in trpγ 1 flies, which did not include a GAL4 knocked into the trpγ gene ( Fig. 7b ). We found a significant rescue of the mutant phenotype using either neuronal GAL4 tested ( elav-Gal4 and iav-Gal4 ; Fig. 7b ). We partially rescued the gap-crossing phenotype by driving UAS-trpγ expression only in scolopale cells with the nompA-GAL4 ( Fig. 7b ). Consistent with a contribution of trpγ to scolopale function, we found that the vacuolar volume of the scolopale cells was reduced in trpγ 1 ( Supplementary Fig. 3a,b ). Except for the reduced size of the scolopale cells, we did not detect other changes in the ultrastructure of the mutant scolopidia. The scolopale rods, scolopale spaces, the neuron cell bodies, dendrites and the dendritic connection to the cap cell all appeared intact and comparable to wild type ( Supplementary Fig. 3a,c ). Suppression of the trpγ phenotype by mutation of CalX Because TRPγ is a Ca 2+ -permeable channel, the loss of the TRPγ-dependent Ca 2+ influx might underlie the proprioceptive defects. To address this model, we applied an approach that we used previously to show that the retinal degeneration in fly photoreceptor cells that resulted from loss of the TRP channel, was due to a decrease in light-dependent Ca 2+ influx. Specifically, we showed that the loss of either TRP or the only Na + /Ca 2+ exchanger (CalX) expressed in flies caused retinal degeneration [40] , [41] . However, the retinal degeneration was much less severe in the double mutant [40] , [41] . Therefore, we wondered whether we could suppress the trpγ 1 gap-crossing phenotype by introducing the calx B mutation, since we found that CalX antibodies (α–CalX) [41] stained neurons and scolopale cells of the wild-type FCO (white dashed outline; Fig. 7c ). The specific labelling in wild type was absent in the calx B FCO (white dashed outline; Fig. 7c ), although there was some background staining, especially of the cuticle (cu; Fig. 7c ). In behavioural assays, loss of CalX alone ( calx B ), caused a gap-crossing deficit, similar to that displayed by trpγ mutant flies ( Fig. 7d ; wild type, 63.5±4.2%, mean±s.e.m. ; trpγ 1 , 11.6±5.9%; calx B , 12.2±8.8%). However, when we introduced the calx B mutation in a trpγ mutant background, the defect in gap-crossing ability was suppressed significantly, as it was less severe than that exhibited by either single mutant alone ( Fig. 7d ; trpγ 1 ; calx B , 42.8±3.3%). TRPγ was activated by membrane stretch in vitro The contribution of TRPγ to fine motor control raises the possibility that TRPγ a mechanically sensitive channel. The activities of mechanically sensitive channels are typically enhanced by membrane stretch [42] . To investigate whether TRPγ might be sensitive to membrane stretch, we expressed TRPγ in HEK293 cells and performed whole-cell patch-clamp recordings. We first tested whether macroscopic TRPγ currents were enhanced by bathing the cells in hypoosmotic (210 mOsm) media. When we performed the recordings under isotonic (300 mOsm) conditions, there was a constitutive, strongly outwardly rectifying conductance ( Fig. 8a,b ), consistent with previous findings [26] , [43] . On exchanging the external media with a hypoosmotic (210 mOsm) bath solution, the current increased threefold ( Fig. 8a–d ). We blocked this activity with Gd 3+ ( Fig. 8a ), an inhibitor of TRPγ [26] , [43] . The current began to increase within 30 seconds, after switching from 300 to 210 mOsm media, and peaked between ∼ 1 to 4 min, depending on the experiments (closed squares, Fig. 8b ). We did not detect a constitutive or hypoosmotic-induced current in mock-transfected cells (open circles, Fig. 8b ). Many TRPC channels are activated through phospholipase C (PLC) signaling cascades. However, addition of a PLC blocker (U73122) did not affect the hypoosmotic induced TRPγ currents ( Fig. 8e ), suggesting that the hypotonicity impacted on TRPγ activation through membrane stretch rather than stimulation of PLC signalling. 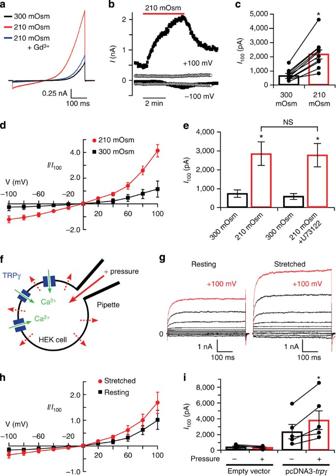Figure 8: TRPγ is activated by membrane stretchin vitro. (a) Overlay of current traces showing the effects of hypoosmotic solution and 100 μm Gd3+on recombinant TRPγ in HEK cells. Current was evoked with a voltage ramp from −100 to 100 mV from a holding potential of −10 mV. (b) Time course of hypoosmotic stimulus on TRPγ currents. Outward and inward macroscopic currents were measured at +100 and −100 mV, respectively, in representative transfected (black squares) and untransfected (open circles) HEK cells. (c) Graph of paired current measurements showing the effects of hypoosmotic stimulus on macroscopic TRPγ currents in HEK cells. Data bars are presented as mean±s.e.m.,n=10. Paired two-tailedt-test, *P≤0.05. (d) Current–voltage (I–V) curves for HEK cells expressing recombinant TRPγ in isoosmotic (black squares) and hypoosmotic (red circles) solutions. Data are presented as mean±s.e.m.,n=10. (e) Summary graph showing the effect of hypoosmotic solution on TRPγ currents in the presence and absence of a PLC inhibitor U73122 (5 μM). Data bars are presented as mean±s.e.m.,n=10. Paired two-tailedt-test, *P≤0.05. (f) Cartoon depicting the activation of TRPγ by membrane stretch induced by positive pipette pressure in a whole cell configuration. (g) Overlay of current traces showing the effects of pressure-induced membrane stretch on the activities of TRPγ recorded from the same HEK cell. Current was evoked with voltage steps from −100 to 100 mV from a holding potential of −60 mV. (h)I–Vcurves for HEK cells expressing recombinant TRPγ under resting (black squares) and stretched (red circles) conditions. Data are presented as mean±s.e.m.,n=5. (i) Graph of paired current measurements showing the effects of pressure-induced membrane stretch on macroscopic currents recorded from HEK cells transfected with either pcDNA3-trpγor an empty vector. Data bars are presented as mean±s.e.m.,n=5. Paired two-tailedt-test, *P≤0.05. Figure 8: TRPγ is activated by membrane stretch in vitro . ( a ) Overlay of current traces showing the effects of hypoosmotic solution and 100 μm Gd 3+ on recombinant TRPγ in HEK cells. Current was evoked with a voltage ramp from −100 to 100 mV from a holding potential of −10 mV. ( b ) Time course of hypoosmotic stimulus on TRPγ currents. Outward and inward macroscopic currents were measured at +100 and −100 mV, respectively, in representative transfected (black squares) and untransfected (open circles) HEK cells. ( c ) Graph of paired current measurements showing the effects of hypoosmotic stimulus on macroscopic TRPγ currents in HEK cells. Data bars are presented as mean±s.e.m., n =10. Paired two-tailed t -test, * P ≤0.05. ( d ) Current–voltage ( I – V ) curves for HEK cells expressing recombinant TRPγ in isoosmotic (black squares) and hypoosmotic (red circles) solutions. Data are presented as mean±s.e.m., n =10. ( e ) Summary graph showing the effect of hypoosmotic solution on TRPγ currents in the presence and absence of a PLC inhibitor U73122 (5 μM). Data bars are presented as mean±s.e.m., n =10. Paired two-tailed t -test, * P ≤0.05. ( f ) Cartoon depicting the activation of TRPγ by membrane stretch induced by positive pipette pressure in a whole cell configuration. ( g ) Overlay of current traces showing the effects of pressure-induced membrane stretch on the activities of TRPγ recorded from the same HEK cell. Current was evoked with voltage steps from −100 to 100 mV from a holding potential of −60 mV. ( h ) I – V curves for HEK cells expressing recombinant TRPγ under resting (black squares) and stretched (red circles) conditions. Data are presented as mean±s.e.m., n =5. ( i ) Graph of paired current measurements showing the effects of pressure-induced membrane stretch on macroscopic currents recorded from HEK cells transfected with either pcDNA3- trpγ or an empty vector. Data bars are presented as mean±s.e.m., n =5. Paired two-tailed t -test, * P ≤0.05. Full size image To test if TRPγ could be activated directly by membrane stretch, we applied positive pressure to HEK293 cells in the whole-cell configuration through the recording pipet ( Fig. 8f ) [44] . We found that repeated pressure stimulations between +30 to 300 mm Hg, starting from a resting pressure of −10 mm Hg, enhanced the current in TRPγ-expressing cells ( Fig. 8g–i ). Moreover, hypoosmotic stimuli or mechanical pressure steps enhanced the conductance in every patched cell that displayed constitutive TRPγ activity ( Fig. 8c,i ). In humans, motor control is categorized into two major types—gross motor skills, required for large body movements such as sitting upright or waving an arm, and fine motor skills, necessary for small precise movements such as picking up and manipulating objects [45] . In Drosophila, gross motor coordination is essential for the large rhythmic movements of the body and limbs during general locomotion (walking), while fine motor coordination is critical for making small changes in the angles and positions of the body and appendages to complete difficult tasks, such as righting or navigating gaps in a terrain. Three Drosophila TRP channels are expressed in proprioceptive organs (Iav, Nan and NOMPC) and elimination of any of these proteins have severe effects on locomotion and gravity sensation [17] , [22] , [23] , [24] . Owing to the major locomotor deficits resulting from the loss of any of these channels, fine motor control is also profoundly affected. Before the current study, it was unclear whether there existed cation channels that contribute exclusively to highly coordinated movements of the body and appendages. In principle, it was possible that the two types of motor coordination depended on the same repertoire of channels (for example, Iav and Nan), and that null mutations would strongly impair all types of coordinated movements, while hypomorphic mutations would affect fine motor control only. We found that TRPγ was required exclusively for fine motor behaviours. In high-frame rate video analysis, both wild-type and trpγ flies traversed the catwalk at a relatively fixed maximum speed, although the trpγ mutants walked more slowly and displayed decreased precision in their leg placements. However, the trpγ mutants used consistently shortened steps, which differed from the abnormally long and highly variable step lengths exhibited by nan mutants [11] . The impairments in fine motor control exhibited by trpγ flies compromised their ability to cross challenging gap sizes. While the mutant animals negotiated gaps of up to 3.0 mm as well as wild type, they were ineffective in traversing larger gaps. This defect was not due to smaller flies, since the lengths of the trpγ bodies were similar to wild-type animals. We propose that the impairment in gap-crossing arises from the inability of the mutants to precisely sense their body position and make the fine postural adjustments required to complete the task. Indeed, the trpγ flies were unable to increase their body angles towards the horizontal position, even as they made successive leg-over-head sweeps. Consequently, they could not fully extend the reach of their front legs to bridge the gap. In sharp contrast, nan and iav mutants were not able to effectively cross even short gaps that virtually all trpγ and wild-type flies were able to negotiate. The majority of work on Drosophila proprioceptive organs has focused on the contribution of the mechanosensory neurons to motor control [17] , [20] , [22] , [23] Unexpectedly, we found that TRPγ was expressed and functioned in both neurons and in glial support cells, called scolopale cells. However, the requirement for TRPγ in neurons appeared to be more significant. RNAi knockdown of trpγ in neurons induced a gap-crossing deficit nearly as severe as the null mutations, while RNAi knockdown of trpγ in scolopale cells, caused a more modest effect. Moreover, we rescued the gap-crossing impairment exhibited by trpγ to a greater extent after re-introducing the wild-type transgene in neurons than in scolopale cells. When we assayed the effects of the trpγ mutation on the leg motor circuit, using EMGs, we rescued the deficit in sensitivity only after expressing the wild-type transgene in neurons. Nevertheless, TRPγ has a dual role in both neurons and scolopale cells, and this is an additional feature that distinguishes TRPγ from TRPs that function in gross motor control. In neurons, the spatial distribution of TRPγ is different from that of Iav, Nan and NOMPC, consistent with the distinct roles of these channels in promoting fine and gross motor control, respectively. In contrast to the cilia-restricted localizations of Iav, Nan, and NOMPC [22] , [46] , we detected TRPγ throughout the neuronal cell bodies and dendrites. We propose that TRPγ functions in chordotonal neurons to sense joint movements needed for fine motor control. In support of this proposal, TRPγ was activated directly by membrane stretch in vitro , and expressed in the dendrites. Furthermore, the TRPγ-dependent Ca 2+ -influx contributes to function, since we suppressed the severity of the behavioural phenotype by eliminating the Na + /Ca 2+ -exchanger, CalX. An additional question concerns the potential role of TRPγ in the scolopale cells. We found that the extensive vacuole network of the mutant scolopale cells in the FCO was reduced in size compared with the wild-type. Various mechanosensors contribute to maintaining vacuolar structures in cells [47] , [48] and growing evidence suggests that TRP channels play critical roles in regulating cell size and shape [49] . This raises the possibility that TRPγ plays a similar role in these support cells, which in turn helps maintain the structural stability of the mechanosensory organs. In summary, we employed high-frame rate video microscopy of fly locomotive behaviours to identify a requirement for a mechanosensitive TRP channel, TRPγ, for fine motor control. The demonstration that a Drosophila channel functions specifically to promote precise body movements raises the question as to whether there exist mechanosensitive Ca 2+ -permeable channels in mammals that are uniquely required for fine motor control. Fly stocks All fly stocks were maintained under standard laboratory conditions under a 12-h light/12-h dark cycle at 25°C. Wild type control flies were Canton S flies, which we backcrossed for 10 generations to w 1118 . We selected w + progeny after each cross, to create the w CS control flies. The pyrexia-Gal4 , nompA-Gal4, and atonal-Gal4 lines were provided by D. Eberl [33] , [39] . The UAS-trpγ RNAi line was from the Vienna Drosophila Resource Center (transformant ID 107656). Df(2l)ED1109, UAS-dsRed , UAS-mCD8::GFP , UAS-2xeGFP , elav-Gal4 , iav-Gal4 , nan-Gal4 , nompC-Gal4 , iav 1 , nan 36a , trp 343 and trpl MB03075 were from the Bloomington Stock Center (Bloomington, IN). We described the calx B mutant previously [41] . Generation of trpγ 1 and trpγ G4 by homologous recombination We generated the trpγ 1 and trpγ G4 mutants by ends-out homologous recombination [28] . To create trpγ 1 , we deleted 180 nucleotides, encoding amino acids 607 to 667, and introduced the white gene at the site of the deletion. To generate trpγ G4 , we replaced 547 nucleotides that including the first two ATGs at the translation start site of trpγ , with a GAL4 gene, which was flanked by the white gene. To generate the pw35- trpγ 1 construct, we amplified 3.38 and 3.04 kb trpγ genomic fragments by PCR and subcloned them into the NotI site and the BamHI sites, respectively, of the pw35 vector [28] . The primers for generating the 3.38-kb fragment were: 5′-ATTTGCGGCCGCATCAACTTATTTCGGTGGGATACTTAC-3′ and 5′-ATTTGCGGCCGCACTTATGTAGTATGCGATTCGATTATTG-3′. The primers for PCRing the 3.04-kb fragment were 5′-GAAGATCTAAGAGGGTTTGTGTGGTTTCGAATAAAC-3′ and 5′-GAAGATCTTTCGCTTTGTTGGCTTGCATGTCTTTAGT-3′. To generate pw35 Gal4 - trpγ G4 , we PCR amplified 3.42 and 2.98 kb trpγ genomic fragments, which we inserted between the BamHI/Acc65I sites and the NotI/SacII sites of the pw35 GAL4 vector, respectively [50] . The primers for amplifying the 3.42-kb fragment were: 5′-CGGGTACCTGCTGTGACGCTAAGGGATTAATAT-3′ and 5′-CGGGATCCTTTCTTTCGGTGTATTTCTCTGTA-3′. The primers for amplifying the 2.98-kb fragment were 5′-TCCCCGCGGTATTCCTGCTGTGGCGAGTTCTGCGCAT-3′ and 5′-ATTTGCGGCCGCCATGATGTGCGATGTGGCTGTGATGA-3′. We introduced pw35- trpγ 1 and pw35 Gal4 - trpγ G4 into w 1118 flies by germline transformation. We generated homologous recombinants as described [28] , and verified the mutations by PCR. We backcrossed trpγ 1 and trpγ G4 for 10 generations to the w 1118 background before conducting the behavioural analyses. Generation of UAS-trpγ and gtrpγ transgenic lines To generate UAS-trpγ flies, we PCR amplified the trpγ coding sequence from w 1118 genomic DNA, which we subcloned between the NotI and the XbaI sites of pUAST [51] . We introduced pUAST- trpγ DNA into w 1118 embryos via germline transformation (BestGene Inc., Chino Hills, CA), and recovered transformant lines with insertions in chromosome 2 and 3. To generate the trpγ genomic transgene ( gtrpγ ), we used P[acman] BAC CH322-162M11 (ref. 52 ), which covers the entire trpγ genomic region and truncates the 5’ and 3’ genes. We inserted P[acman] BAC CH322-162M11 by ΦC31-mediated transgenesis (Rainbow Transgenic Flies Inc., Camarillo, CA) into the VK00033 attP site on chromosome 3l (Bloomington stock #24871) [52] , [53] . TRPγ antibodies A TRPγ peptide (amino acids 1,065–1,085) was injected into rabbits to raise polyclonal antibodies (Covance Inc.). This sequence was unique among Drosophila proteins. We affinity purified the TRPγ antibodies (α–TRPγ) from whole serum using the synthesized peptide immobilized on an Affi-Gel 10 (Bio-Rad) column. High-pressure freezing and electron microscopy We dissected Drosophila legs from 3–5-day-old male flies, and transferred them to yeast paste containing 10% methanol, or hexadecene, which served as a cryoprotectant [54] . The samples were then freeze substituted in a fixing cocktail containing 2% osmium and 0.2% uranyl acetate in acetone and 5% water for better preservation of membranes [55] . We performed the freeze substitution in a Leica EM AFS 2/FSP with a modified schedule (correspondence Rick Fetter, Janelia Farms HHMI). We incubated the samples at −90 °C for 72 h, brought them to −25 °C with a slope of 5 °C per h, and then held them at −25 °C for 17 h to increase membrane contrast [56] . Samples were then sloped 5 °C per h to 4 °C and held there for further processing. After three acetone rinses, we gradually infiltrated the samples at 25 °C with a mixture of Eponate 12 and Spurr’s resin (1:1, Ted Pella) with acetone, 25% for 2 h, 50% for 2 h, and 75% overnight. After three exchanges with 100% resin, we cured the samples at 60 °C for 2 days. We oriented the blocks and cut longitudinal and cross sections through the FCO on a Reichert Ultracut E with a Diatome Diamond knife. Sections (60 nm) were picked up on formvar coated 1 × 2 mm copper slot grids and stained with 2% uranyl acetate and 0.3% lead citrate. Grids were viewed on a Phillips CM 120 transmission EM operating at 80 kV and digital images were captured with an ER-80 AMT 8 megapixel CCD camera. Immunostaining Leg samples were high-pressure frozen as above, but were freeze substituted with a low temperature protocol utilizing Lowicryl HM20 resin (Polysciences #15924). Samples were freeze-substituted with fixing cocktail containing 0.2% uranyl acetate (in methanol), 0.2% glutaraldehyde in acetone with 5% water. We held the legs at −90 °C for 32 h, and then increased the temperature to −45 °C with a slope of 4 °C per h. We gradually infiltrated the samples at −45 °C with a mixture of HM20 resin with acetone, 50% for 1.5 h, 75% for 1.5 h, 100% for 1.5 h and finally overnight after a fresh exchange of 100% resin. Embedded samples were cured under ultraviolet light for 24 h at −45 °C, and then incubated for 24 h at room temperature before cutting. We trimmed and oriented the resin blocks, and cut serial 0.5-μm longitudinal sections through the femoral leg segment and the FCOs. We treated the sections with 50 mM glycine for 10 min at room temperature and blocked the sections overnight at 4 °C in TBS (50 mM Tris-Cl,150 mM NaCl, pH 7.5) containing 10% BSA (Sigma). For staining with anti-TRPγ, we incubated the sections with primary rabbit TRPγ antibodies diluted 1:200 in TBS-T (50 mM Tris-Cl, 150 mM NaCl, 0.05% Tween-20, pH 7.5) for 72 h at 4 °C, washed with TBS and incubated overnight in TBS-T at 4 °C. For staining with α–CalX, we incubated the sections with primary rabbit CalX antibodies [41] diluted 1:200 in TBS-T overnight at 4 °C, washed with TBS and incubated overnight in TBS-T at 4 °C. Sections probed with α–TRPγ and α–CalX were subsequently incubated in secondary antibodies (Alexa Fluor 488F(ab′) 2 fragment of goat anti-rabbit IgG; A11070, Life Technologies) diluted 1:500 in TBS for 1 h at room temperature, washed with TBS, incubated overnight in TBS at 4 °C and sealed under glass cover slips with Vectashield mounting media with DAPI (4′,6-diamidino-2-phenylindole). We viewed the sections using a Zeiss LSM700 and processed the images with Zen software (Carl Zeiss Microscopy). Monitoring activities using actometers We transferred individual 4-day-old male flies into recording tubes containing 1% agarose with 5% sucrose, and monitored locomotor activities using the Drosophila Activity Monitoring system (Trikinetics Inc., Waltham, MA). We binned the number of activity events per individual fly every 30 min. Negative geotaxis assay We transferred 30 male flies (3–5 days old) to a 100-ml graduated cylinder, sharply tapped the cylinder down three times and recorded videos (30 fps) of the flies ascending the sides of the cylinders. The climbing index is the percentage of flies that climbed past a line 10 cm from the bottom of the cylinder in 10 s. Righting reflex assay We introduced 30 male flies (3–5 days old) to a 100-ml graduated cylinder, and tapped the flies to the bottom as described for the negative geotaxis assay. We positioned a video camera with a macro lens so that it could record the bottom surface of the cylinder (30 fps). After each set of taps, 0–5 flies fell on their backs and performed the righting reflex. Each group of 30 flies was tapped and recorded a maximum of five times. New groups of flies were then tested until the total number of observed righting reflexes was >100 per genotype. We analysed the videos frame-by-frame to determine the elapsed time for completing the reflex. Recording apparatus for analysis of locomotion behaviours We recorded locomotion behaviour at 200–250 frames per second (fps), and at a resolution of 1,280 × 1,024 pixels using a pco.1200s digital 10-bit CMOS camera system (PCO AG, Germany). A 3.3 × macro zoom lens (NT56–524, Edmund Optics, Barrington, NJ) provided a 6.4–21.3 mm field of view on the 0.5′ sensor at a working distance of 90 mm. We mounted the camera orthogonally to a circular recording chamber (10 cm in diameter using optomechanical components from Thorlabs Inc., Newton, NJ). The recording chamber was surrounded by 10 cm high white paper to reduce the influences of external visual stimuli, and was illuminated by an adjustable intensity array of 126 white LEDs behind a diffuser (CN-160 and CN-AC2, Amazon.com). The chamber accommodated a 34 × 10 × 4 mm walking platform (with or without a central gap) made of black Delrin acetal resin. To obtain better contrast in the video recordings, we placed a pair of additional spotlights at both ends of the platform 10 cm away and 60° incident to the top surface. To prevent the flies from escaping, we surrounded the walking platform with 0.5 cm of water. To allow for precise positioning of the platform in the cameras field of view, we mounted the entire recording chamber on top of a three-axis flexure stage (MBT616D, Thorlabs Inc.). Catwalk assay We performed the assays using male flies with blinded genotypes. We cut the wings of the flies (3–5 days old) to ∼ 1/4 their original length under ice anaesthesia, and then recorded the flies walking behaviour over a gapless platform at 250 fps. We collected three videos per fly, and five flies per genotype. Of the three recordings per fly, we chose the single video in which the fly exhibited the ‘straightest’ crossing (no turns and/or stops as determined by slow motion analysis) for the tracking analysis. We tracked the frame-by-frame position of each leg tip using the MTrackJ plugin [57] in ImageJ [58] . Gap-crossing assay The gap-crossing assay, which we performed using blinded genotypes, was similar to that described previously [12] . In brief, we cut the wings of 3–5-day-old male flies to ∼ 1/4 their original length under ice anaesthesia, and recorded their ability to cross gaps of various widths (1.0–4.0 mm) at 250 fps. We chose a 3.5 mm gap for the screening since this was a challenging but achievable width for wild type. To screen for gap-crossing proficiency (successful or unsuccessful), we recorded the first 10 crossing attempts for each fly. We tested 10 flies per genotype. The percentage of successful crossings represents the aggregate performance of 10 files in 100 total crossing attempts. During the screening, we recorded a small number of videos for each genotype to determine the body lengths. To perform the detailed kinematic analyses during the gap crossings, we collected three videos for each fly, and recorded five flies per genotype. To perform the tracking analyses, we chose a single video for each fly, based on the ‘straightest’ crossing (orthogonal to the camera view as determined by slow motion analysis). We tracked the frame-by-frame position of each front leg tip, head position and tail position using the MTrackJ plugin [57] for ImageJ [58] . Extracellular recordings We performed electromyogram recordings of excitatory junction potentials from fly leg extensor muscles in response to tibia flexion as previously described [36] , [37] . In brief, we decapitated 3–5-day-old male flies under ice anaesthesia, and allowed them to recover for 1 h in a humidified chamber. If the flies were able to stand and walk, we mounted them for the recordings with their dorsal side up, and on the edge of a waxed cover slip so that the tibial segment of one leg was able to hang over the edge. The distal end of the femur was secured with wax. Tibia flexion was stimulated by sinusoidal displacement of a wire loop attached to the cone of a loudspeaker (273-092, RadioShack.com). A 2-Hz sine wave from a signal generator (Velleman PCGU1000, Allspectrum.com) resulted in ∼ 20° of tibia movement about the femoral joint. We performed multiple sets of tibia flexion movements (10 movements per set), with each set spaced 1 min apart to minimize habituation. We performed each recording with a 0.5–1-MΩ borosilicate electrode using an IE-210 intracellular electrometer (Warner Instruments LLC, Hamden, CT). Digital acquisition was performed using a PowerLab 4/30 DAQ with analysis in LabChart 5 (ADInstruments Inc., Colorado Springs, CO). Cell culture We cultured HEK293 cells (ATCC) in DMEM medium supplemented with 10% fetal bovine serum and 1% penicillin/streptomycin at 37 °C in a humidified atmosphere of 5% CO 2 . Cells were plated onto glass coverslips coated with poly L -lysine for 24 h before transfection. Split cells were co-transfected with plasmids encoding pcDNA3-TRPγ or empty pcDNA3.1 (mock) with GFP (1 and 0.5 μg, respectively) for 6–24 h using either Polyfect or Lipofectamine LTX reagents (Qiagen, Valencia, CA or Life Technologies, Grand Island, NY). Patch-clamp recordings We collected whole-cell current recordings of TRPγ in HEK293 cells under voltage-clamp conditions. Macroscopic TRPγ currents were evoked using voltage ramps or steps of 500 ms duration from –100 to 100 mV from a holding potential of −10 mV. For hypoosmotic stimulation, we used two different extracellular bath solutions: (1) an isotonic (300 mOsm) solution containing (in mM) 90 NaCl, 100 D -mannitol, 5 KCl, 2 MgCl 2 , 2 CaCl 2 , 10 HEPES, 10 D -glucose, pH 7.4 adjusted with NaOH; and (2) a hypotonic (210 mOsm) solution prepared by reducing the final concentration of D -mannitol to 10 mM without changing the ionic composition of the solution. The pipette solution was (in mM) 135 CsCl, 2 MgCl 2 , 10 HEPES, 5 EGTA, 5 Na 2 -ATP, pH 7.2 adjusted with CsOH. Pressure stimulation was applied via a 100-ml syringe placed in line with a pressure manometer (SYS-PM100R, World Precision Instruments Inc., Sarasota, FL) connected to the pressure port of the pipette microelectrode holder. Positive pressure steps of between +30 to +300 mm Hg were applied from a resting pressure of −10 mm Hg. Pressure was held constant via actuation of an in-line stopcock during the recordings. Macroscopic currents were acquired using an Axopatch 200B (Axon Instruments) patch clamp amplifier interfaced via a Digidata 1440A (Molecular Devices) to a PC running the pClamp 10.4 suite of software (Molecular Devices). Macroscopic currents were filtered at 1 kHz and digitized at 2 kHz. Whole-cell capacitance and series resistances were routinely compensated. Only recordings where access resistance and capacitance changed <10% over the course of the experiment were used. How to cite this article: Akitake, B. et al. Coordination and fine motor control depend on Drosophila TRPγ. Nat. Commun. 6:7288 doi: 10.1038/ncomms8288 (2015).